A statin-loaded reconstituted high-density lipoprotein nanoparticle inhibits atherosclerotic plaque inflammation Inflammation is a key feature of atherosclerosis and a target for therapy. Statins have potent anti-inflammatory properties but these cannot be fully exploited with oral statin therapy due to low systemic bioavailability. Here we present an injectable reconstituted high-density lipoprotein (rHDL) nanoparticle carrier vehicle that delivers statins to atherosclerotic plaques. We demonstrate the anti-inflammatory effect of statin-rHDL in vitro and show that this effect is mediated through the inhibition of the mevalonate pathway. We also apply statin-rHDL nanoparticles in vivo in an apolipoprotein E-knockout mouse model of atherosclerosis and show that they accumulate in atherosclerotic lesions in which they directly affect plaque macrophages. Finally, we demonstrate that a 3-month low-dose statin-rHDL treatment regimen inhibits plaque inflammation progression, while a 1-week high-dose regimen markedly decreases inflammation in advanced atherosclerotic plaques. Statin-rHDL represents a novel potent atherosclerosis nanotherapy that directly affects plaque inflammation. Atherosclerotic diseases, such as acute myocardial infarction, are a major cause of death and disability worldwide ( http://www.who.int/cardiovascular_diseases/en/ ). Preventive strategies currently focus on controlling risk factors, such as smoking, blood pressure, serum glucose and lipid levels [1] . Despite the success of these preventive measures, substantial residual risk remains even when treatment goals are fully met [2] . In patients who suffered a myocardial infarction, the recurrence risk of an acute coronary syndrome is high, particularly within the first year when recurrence rates are up to 17.4% (ref. 3 ). A recent study explained this phenomenon by showing that a systemic response to ischaemic injury aggravates inflammation in atherosclerotic plaques at a distance because of increased monocyte (Mo) recruitment [4] . Mos that infiltrate the plaque differentiate into macrophages (MΦs), which produce proteolytic enzymes that digest extracellular matrix causing plaque rupture [5] . The immediate site of plaque rupture contains a high concentration of inflammatory cells [6] . Plaque inflammation is therefore pursued as a therapeutic target to prevent atherothrombotic events [7] . In the current study, we developed a nanomedicine-based delivery strategy based on reconstituted high-density lipoprotein (rHDL) nanoparticles that allow for drug delivery to atherosclerotic plaques. As a cargo for our rHDL nanoparticles we selected a 3-hydroxy-3-methylglutaryl coenzyme A reductase (HMGR) inhibitor, or statin. Statins are widely orally prescribed serum low-density lipoprotein (LDL) cholesterol-lowering drugs that upregulate LDL receptor expression in hepatocytes [8] . In addition to its effect on hepatocytes, various studies have established the potent immunomodulating effects of HMGR inhibition in inflammatory cells [9] , [10] , [11] . In an atherosclerotic mouse model in which statins did not affect lipid levels, reduced plaque formation was shown with extremely high doses of oral statin therapy [12] . However, in humans increasing the oral statin dose to attain higher plasma concentrations is not feasible because of the dose-dependent onset of adverse effects such as hepatoxicity and myopathy [13] . Normal doses of orally ingested statins hardly enter the systemic circulation as biotransformation occurs in the liver [14] . We addressed this issue by developing a statin-loaded rHDL nanoparticle ([S]-rHDL) that can be administered intravenously, can augment bioavailability and can facilitate the delivery of statins to atherosclerotic plaque. We show, in an apolipoprotein E-knockout (apoE-KO) mouse model of atherosclerosis, that a 3-month low-dose- as well as a 1-week high-dose [S]-rHDL treatment regimen markedly reduces plaque MΦ content. Study summary A schematic overview of the study design is shown in Fig. 1 . First, we studied the characteristics of [S]-rHDL and its efficacy in different cell lines in vitro . Subsequently, biodistribution and toxicity, as well as uptake by atherosclerotic plaque MΦs, were investigated in mouse models in vivo . Next, we investigated the in vivo efficacy of a low-dose long-term [S]-rHDL infusion regimen on plaque development and a short-term high-dose infusion regimen on plaque regression in apoE-KO mice. 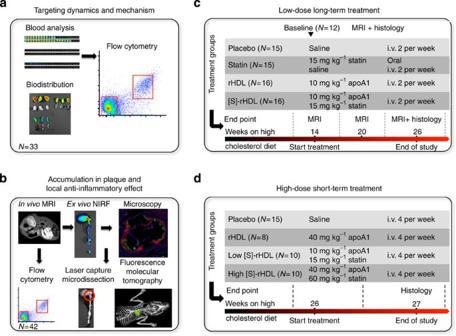Figure 1: Schematic of the study design. (a) The targeting dynamics, targeting mechanism and anti-inflammatory action of [S]-rHDL in apoE-KO mice were investigated by analysing the dynamics of phospholipids and hydrophobic cargos of [S]-rHDL in the blood using NIRF and flow cytometry. The biodistribution was evaluated in organs with NIRF. (b) Magnetic resonance imaging, NIRF, fluorescence microscopy and flow cytometry were used to validate the plaque macrophage-targeting efficiency of [S]-rHDL. The effect of [S]-rHDL on the mRNA levels of inflammatory genes of plaque macrophages was determined in macrophages isolated with laser capture microdissection. Fluorescence molecular tomography and computed tomography were used to assess the effect of [S]-rHDL on inflammatory protease activity in aortic root plaques. (c) The efficacy of low-dose long-term (12 weeks) [S]-rHDL treatment on disease progression was evaluated in the abdominal aortas with MRI and in aortic roots with histology. (d) The efficacy of high-dose short-term (1 week) [S]-rHDL treatment was evaluated in aortic roots with histology. Figure 1: Schematic of the study design. ( a ) The targeting dynamics, targeting mechanism and anti-inflammatory action of [S]-rHDL in apoE-KO mice were investigated by analysing the dynamics of phospholipids and hydrophobic cargos of [S]-rHDL in the blood using NIRF and flow cytometry. The biodistribution was evaluated in organs with NIRF. ( b ) Magnetic resonance imaging, NIRF, fluorescence microscopy and flow cytometry were used to validate the plaque macrophage-targeting efficiency of [S]-rHDL. The effect of [S]-rHDL on the mRNA levels of inflammatory genes of plaque macrophages was determined in macrophages isolated with laser capture microdissection. Fluorescence molecular tomography and computed tomography were used to assess the effect of [S]-rHDL on inflammatory protease activity in aortic root plaques. ( c ) The efficacy of low-dose long-term (12 weeks) [S]-rHDL treatment on disease progression was evaluated in the abdominal aortas with MRI and in aortic roots with histology. ( d ) The efficacy of high-dose short-term (1 week) [S]-rHDL treatment was evaluated in aortic roots with histology. Full size image [S]-rHDL characteristics We constructed [S]-rHDL from human apolipoprotein A-1 (ApoA1), the phospholipids 1-myristoyl-2-hydroxy-sn-glycero-phosphocholine and 1,2-dimyristoyl-sn-glycero-3-phosphatidylcholine, in which lipophilic simvastatin was encapsulated. This resulted in discoid-shaped nanoparticles of 25–30 nm in diameter as determined by dynamic light-scattering and transmission electron microscopy (TEM) ( Fig. 2a , Supplementary Fig. 1 , and Supplementary Table 1 ). Its exact composition was established by phosphate determinations and simvastatin measurements using high-performance liquid chromatography (HPLC) ( Supplementary Table 1 ). Stability experiments with the free drug and the [S]-rHDL nanoparticle formulation in mouse serum demonstrated the protective function of the rHDL nanoparticle towards statin degradation ( Supplementary Fig. 2 ). To allow its visualization in cells and tissues via imaging techniques, we also synthesized a variant in which an amphiphilic magnetic resonance imaging (MRI) contrast agent, gadolinium–diethylene triamine pentaacetic acid–distearyl amide and/or fluorescent dyes (Cy5.5, DiO or DiR) were incorporated ( Fig. 2a ). 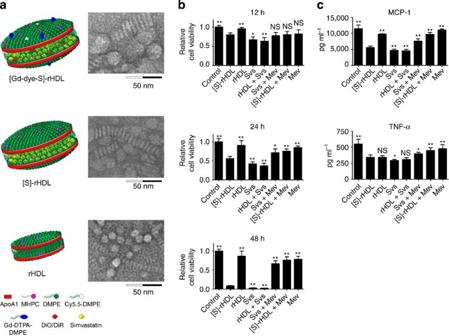Figure 2: Schematic representations of the nanoparticle formulations andin vitroefficacy data. (a) Schematic representation of dual gadolinium and fluorescent dye (Cy5.5, DiO, DiR)-labelled statin containing reconstituted high-density lipoprotein ([Gd-dye-S]-rHDL), [S]-rHDL and rHDL. Negative staining TEM images of each of the aforementioned particles showed the typical disk-like morphology. The circular shapes are nanoparticles vieweden face, while the striped configurations are rouleaux of nanoparticles viewed from the side. Dynamic light-scattering measurements showed the average size of [Gd-dye-S]-rHDL to be 28.5 nm, of [S]-rHDL to be 26.0 nm and of rHDL to be 10.5 nm. For larger view TEM also seeSupplementary Fig. 1. (b)In vitrocell viability assays of murine macrophages (J774A.1), incubated with combinations of [S]-rHDL (10 μM statin), free simvastatin (10 μM), rHDL plus-free statin (10 μM), free statin (10 μM) plus mevalonate (100 μM), [S]-rHDL (10 μM) plus mevalonate (100 μM) and only mevalonate (100 μM). There was also a control group of cells not incubated with anything. Macrophage cell viability is markedly decreased in the [S]-rHDL and free statin group. This effect is abolished by addition of mevalonate, indicating that the effect of HMGR inhibition on cell viability is mediated through the mevalonate pathway.N=6 for all bars. (c) Production of the inflammatory cytokines MCP-1 and TNF-α. Lipopolysaccharide (LPS)- and INF-γ-challenged macrophages were incubated with the same treatments as mentioned above for 24 h. MCP-1 and TNF-α levels are markedly reduced by [S]-rHDL and free statin. MCP-1 and TNF-α levels are restored by the addition of mevalonate to [S]-rHDL and free statin incubation.N=6 for all bars. Cell viability in the different groups was not affected under these conditions (Supplementary Fig. 4). All error bars are 95% confidence intervals.P-values are calculated with Mann–WhitneyU-tests for comparisons with [S]-rHDL, *P<0.05, **P<0.01. Kruskal–WallisP-values are <0.0001 for all plots. Figure 2: Schematic representations of the nanoparticle formulations and in vitro efficacy data. ( a ) Schematic representation of dual gadolinium and fluorescent dye (Cy5.5, DiO, DiR)-labelled statin containing reconstituted high-density lipoprotein ([Gd-dye-S]-rHDL), [S]-rHDL and rHDL. Negative staining TEM images of each of the aforementioned particles showed the typical disk-like morphology. The circular shapes are nanoparticles viewed en face , while the striped configurations are rouleaux of nanoparticles viewed from the side. Dynamic light-scattering measurements showed the average size of [Gd-dye-S]-rHDL to be 28.5 nm, of [S]-rHDL to be 26.0 nm and of rHDL to be 10.5 nm. For larger view TEM also see Supplementary Fig. 1 . ( b ) In vitro cell viability assays of murine macrophages (J774A.1), incubated with combinations of [S]-rHDL (10 μM statin), free simvastatin (10 μM), rHDL plus-free statin (10 μM), free statin (10 μM) plus mevalonate (100 μM), [S]-rHDL (10 μM) plus mevalonate (100 μM) and only mevalonate (100 μM). There was also a control group of cells not incubated with anything. Macrophage cell viability is markedly decreased in the [S]-rHDL and free statin group. This effect is abolished by addition of mevalonate, indicating that the effect of HMGR inhibition on cell viability is mediated through the mevalonate pathway. N =6 for all bars. ( c ) Production of the inflammatory cytokines MCP-1 and TNF-α. Lipopolysaccharide (LPS)- and INF-γ-challenged macrophages were incubated with the same treatments as mentioned above for 24 h. MCP-1 and TNF-α levels are markedly reduced by [S]-rHDL and free statin. MCP-1 and TNF-α levels are restored by the addition of mevalonate to [S]-rHDL and free statin incubation. N =6 for all bars. Cell viability in the different groups was not affected under these conditions ( Supplementary Fig. 4 ). All error bars are 95% confidence intervals. P -values are calculated with Mann–Whitney U -tests for comparisons with [S]-rHDL, * P <0.05, ** P <0.01. Kruskal–Wallis P -values are <0.0001 for all plots. Full size image In vitro efficacy of [S]-rHDL To assess the therapeutic potential and function of [S]-rHDL, we investigated its anti-inflammatory effect in vitro . First, we investigated the effect of [S]-rHDL on the viability of murine MΦs (J774A.1) as well as on hepatocytes, endothelial cells and smooth muscle cells as a function of incubation concentration and time. Cells were incubated with rHDL or [S]-rHDL, with statin doses of 1, 10 and 100 μM ( Supplementary Fig. 3 ). MΦ survival was comparable in the rHDL- and [S]-rHDL-incubated cells at 6 and 12 h time points, while MΦ survival decreased in the [S]-rHDL-incubated cells at 24 and 48 h. A similar response was observed in cultured endothelial cells. Significantly less loss in cell viability was observed for the smooth muscle cells and hepatocytes ( Supplementary Fig. 3 ). Subsequently, we investigated whether the effect of [S]-rHDL on MΦ cell viability was mediated through the mevalonate pathway. In MΦs incubated with [S]-rHDL or free statin (10 μM), we observed a nearly complete loss of cell viability at 48 h incubation time, while this did not occur in cells incubated with rHDL. This effect was abolished when mevalonate was added to [S]-rHDL or free statin ( Fig. 2b ). Next, we evaluated the effect of [S]-rHDL on the expression of inflammatory cytokines ( Fig. 2c ). We first stimulated the MΦs with lipopolysaccharide and interferon-γ for 16 h. Cell viability at these conditions was not markedly affected. We then treated the cells with different treatments for 24 h under serum-free conditions and assessed expression of the anti-inflammatory markers—Mo chemotactic protein-1 (MCP-1) and tumour necrosis factor-α (TNF-α). We observed a decrease in expression of MCP-1 and TNF-α in MΦs treated with [S]-rHDL or free statins. The expression of MCP-1 and TNF-α was restored by the addition of mevalonate in MΦs treated with [S]-rHDL and free statins ( Fig. 2c ). Cell viability of MΦs treated with [S]-rHDL was similar to control cells ( Supplementary Fig. 4 ). These data show that [S]-rHDL reduces cell viability and the production of inflammatory cytokines by inhibiting the mevalonate pathway. Subsequently, we investigated the mechanism by which [S]-rHDL decreases MΦ cell viability. We observed that [S]-rHDL decreased MΦ proliferation. We also observed that [S]-rHDL causes non-apoptotic MΦ cell death ( Supplementary Fig. 4 ). In vivo biodistribution and toxicity studies To investigate the biodistribution of [S]-rHDL, we designed an [S]-rHDL nanoparticle that carried two labels, namely Cy5.5 conjugated to a phospholipid in the corona and the hydrophobic dye DiO or DiR in its core. Cy5.5–phospholipids were incorporated in the corona, while the hydrophobic dyes DiO and DiR were incorporated in the simvastatin-loaded core of [S]-rHDL ( Fig. 2a ). Lipoproteins, including HDL, are dynamic systems that are known to exchange lipid components [15] , [16] , [17] . Therefore, we hypothesized that the hydrophobic DiO/DiR core label would display a different kinetic behaviour from the amphiphilic phospholipid-Cy5.5 corona label. To investigate this, we injected apoE-KO mice ( N =21) with the dual-labelled [S]-rHDL, killed them at different time points ( N =3 per time point) and collected their blood, hearts, aortas, spleens, livers and kidneys. The blood was separated into three fractions—that is, plasma, mononuclear cells (MNCs) and red blood cells (RBCs). We observed that the majority of the Cy5.5-labelled phospholipids remained in the plasma fraction of the blood, while a small fraction was transferred to the RBCs ( Fig. 3a,b ). The core label DiO was detectable in the serum fraction only and displayed longer circulation kinetics. Further analysis of blood using flow cytometry revealed the small fraction of DiO associated with MNC to be most abundantly present in pro-inflammatory Gr-1 hi Mos ( Fig. 3c , Supplementary Fig. 5 ). 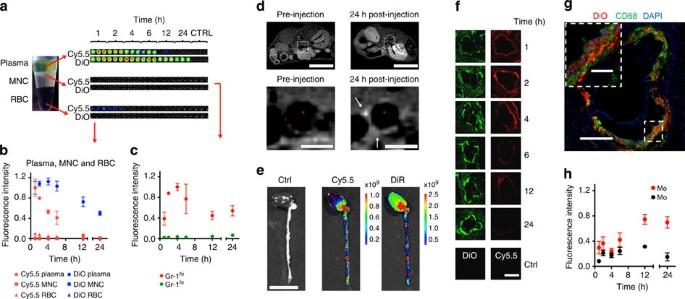Figure 3: Pharmacokinetics and accumulation in plaque of labelled nanoparticles. (a) Cy5.5- and DiO-labelled [S]-rHDL was intravenously injected to apoE-KO mice (N=21, three mice per time point) and blood and tissues were analysed at different time points post injection. NIRF shows that components from the lipid monolayer (Cy5.5) have much shorter blood half-life than components from hydrophobic core (DiO). It also shows that the majority of [S]-rHDL stays in the serum and very little in the RBCs and MNCs. (b) Fluorescence intensity in serum, MNC and RBC is quantified (N=21, three mice per time point). We calculated that plasma half-life of [S]-rHDL is 21.9 h for the DiO signal. (c) Flow cytometric analysis of blood cells shows that [S]-rHDL targets Gr-1hipro-inflammatory Mos more efficiently than Gr-1loanti-inflammatory Mos in the blood (N=21, three mice per time point). (d) Typical T1-weighted 9.4 Tesla magnetic resonance images of the abdominal aorta of an apoE-KO mouse, made at identical locations, before and 24 h after injection of [Gd-Dye-S]-rHDL. The lumen is indicated by *. The scale bar in the upper images represents 10 mm and in the lower images represents 1 mm. The 24-h post-injection image showed signal enhancement in the vessel wall (white arrows), indicative of nanoparticle infiltration and retention in the aortic plaques. (e) [S]-rHDL labelled with Cy5.5 (lipid monolayer) and DiR (hydrophobic core) was intravenously injected into apoE-KO mice. NIRF shows that Cy5.5 and DiR preferentially accumulate in the areas rich in atherosclerotic lesions. The scale bar represents 10 mm. (f) Cy5.5 and DiO both appear in the plaque; until 4 h post-injection the presence of Cy5.5 declines while DiO remains present. The scale bar represents 500 μm. (g) DiO-labelled [S]-rHDL colocalizes in the plaque with CD68 (macrophages). The scale bar in the inset represents 100 μm, and in the overview 400 μm. (h) Flow cytometric analysis of cells in aorta walls shows that [S]-rHDL is taken up by plaque macrophages; furthermore, macrophages are targeted more efficiently than monocytes (N=3 per time point). Figure 3: Pharmacokinetics and accumulation in plaque of labelled nanoparticles. ( a ) Cy5.5- and DiO-labelled [S]-rHDL was intravenously injected to apoE-KO mice ( N =21, three mice per time point) and blood and tissues were analysed at different time points post injection. NIRF shows that components from the lipid monolayer (Cy5.5) have much shorter blood half-life than components from hydrophobic core (DiO). It also shows that the majority of [S]-rHDL stays in the serum and very little in the RBCs and MNCs. ( b ) Fluorescence intensity in serum, MNC and RBC is quantified ( N =21, three mice per time point). We calculated that plasma half-life of [S]-rHDL is 21.9 h for the DiO signal. ( c ) Flow cytometric analysis of blood cells shows that [S]-rHDL targets Gr-1 hi pro-inflammatory Mos more efficiently than Gr-1 lo anti-inflammatory Mos in the blood ( N =21, three mice per time point). ( d ) Typical T1-weighted 9.4 Tesla magnetic resonance images of the abdominal aorta of an apoE-KO mouse, made at identical locations, before and 24 h after injection of [Gd-Dye-S]-rHDL. The lumen is indicated by *. The scale bar in the upper images represents 10 mm and in the lower images represents 1 mm. The 24-h post-injection image showed signal enhancement in the vessel wall (white arrows), indicative of nanoparticle infiltration and retention in the aortic plaques. ( e ) [S]-rHDL labelled with Cy5.5 (lipid monolayer) and DiR (hydrophobic core) was intravenously injected into apoE-KO mice. NIRF shows that Cy5.5 and DiR preferentially accumulate in the areas rich in atherosclerotic lesions. The scale bar represents 10 mm. ( f ) Cy5.5 and DiO both appear in the plaque; until 4 h post-injection the presence of Cy5.5 declines while DiO remains present. The scale bar represents 500 μm. ( g ) DiO-labelled [S]-rHDL colocalizes in the plaque with CD68 (macrophages). The scale bar in the inset represents 100 μm, and in the overview 400 μm. ( h ) Flow cytometric analysis of cells in aorta walls shows that [S]-rHDL is taken up by plaque macrophages; furthermore, macrophages are targeted more efficiently than monocytes ( N =3 per time point). Full size image Near infrared fluorescence (NIRF) imaging and fluorescence microscopy of the spleen, liver and kidneys revealed the highest DiR presence in the liver tissue ( Supplementary Fig. 6 ). Nanoparticles were found in heart, aorta, liver, spleen and kidney tissues but not in the muscle tissue ( Supplementary Fig. 6 ). A combination of restricted nanoparticle accessibility from the muscle microvasculature to muscle tissue and the absence of SR-B1, ABCA-1 or ABCG-1 expression may explain why our nanoparticle was not found to be associated with myocytes. In the spleen, DiR signal colocalized with CD68-stained Mos/MΦs ( Supplementary Fig. 7 ). Flow cytometry analysis of spleen cells revealed that MΦs and Ly-6c hi (Gr-1 hi ) Mos took up [DiO-S]-rHDL most efficiently, while neutrophils and Ly-6c lo (Gr-1 hi ) moncoytes took up markedly less nanoparticles. [S]-rHDL did not exert toxic effects on liver, kidney or myocytes when it was administered to mice at a high dose (60 mg kg −1 simvastatin, 40 mg kg −1 ApoA1, four intravenous (i.v.) infusions per week) for a week ( Supplementary Fig. 8 ). Accumulation and uptake in atherosclerotic plaques To assess whether our nanoparticles accumulated in atherosclerotic lesions and were taken up by plaque MΦs, we conducted two experiments. In the first experiment, apoE-KO mice on a high-cholesterol diet for 28 weeks were infused with gadolinium and statin containing rHDL ([Gd-S]-rHDL, N =3) or placebo ( N =3). In vivo MRI experiments performed with a 9.4 Tesla scanner revealed signal enhancement in the vessel wall on T1-weighted images 24 h after infusion of [Gd-S]-rHDL, indicating pronounced accumulation of our nanoparticle in the vessel wall ( Fig. 2d ). In the second experiment, dual-labelled [S]-rHDL, with Cy5.5–phospholipids in the corona and DiO/DiR in the core, was injected into apoE-KO mice. Twenty-four hours post injection, the mice were killed and their hearts and aortas were excised. The distribution of DiR-labelled [S]-rHDL in intact aortas was investigated by NIRF imaging, which revealed its accumulation in regions rich in plaques ( Fig. 3e ). The targeting kinetics of DiO (the core label) and Cy5.5-phospholipid label displayed a pattern similar to the blood kinetics ( Fig. 3f ), namely that the Cy5.5-labelled phospholipids appeared in the plaque until 4 h post injection, after which their presence declined. In contrast, the DiO core label was retained in the plaque up to at least 24 h. Furthermore, fluorescence microscopy of plaques revealed colocalization of DiO-labelled [S]-rHDL with MΦs in the aortic root ( Fig. 3g ). Flow cytometry of cells from atherosclerotic plaques showed that the fluorescence intensity of the core label DiO was five- to sixfold stronger in MΦs than in freshly recruited Mos ( Fig. 3h , Supplementary Fig. 5 ). In vivo efficacy of low-dose [S]-rHDL infusions To investigate the effect of [S]-rHDL on plaque inflammation we used apoE-KO mice ( N =74) that were on a high-cholesterol diet for 14 weeks in order to develop atherosclerosis. Statins are known not to affect blood cholesterol levels of apoE-KO mice, as they lack the major ligand for the LDL receptor, namely apoE [18] , [19] , and also metabolize statins very rapidly in their livers [20] , making this a suitable model to solely investigate the anti-inflammatory effects of HMGR inhibition. To limit a dominant therapeutic effect of rHDL itself, we used a low ApoA1 dose. While the mice remained on the high-cholesterol diet, they received biweekly infusions of [S]-rHDL (15 mg kg −1 statin, 10 mg kg −1 ApoA1, N =16), placebo (saline infusion, N =15), orally dosed statin (15 mg kg −1 statin daily, N =15) or biweekly infusion of bare rHDL nanoparticles (10 mg kg −1 ApoA1, N =15) for 12 consecutive weeks. We also included a group of mice that were killed when the other groups started their treatment, which we refer to as the baseline group ( N =12). As plaque formation in apoE-KO mice occurs more rapidly in the aortic root than in the abdominal aorta, we were able to study the effects of [S]-rHDL in both early and established atherosclerotic lesions. In the aortic root, plaque formation is reproducible, consistent and homogenous, and covers a length of less than 0.5 mm, which enables us to apply quantitative histology analyses. We evaluated 42 cross-sections of the aortic sinus area per mouse. This resulted in the analysis of 3,108 cross-sections in total. Cross-sections were stained for connective tissue with haematoxylin phloxine saffron (HPS) or immunostained with CD68 antibodies to visualize the MΦs. We developed a quantitative and digitized method with in-house developed software (Matlab) for the analysis of the histology images, to quantify total plaque area (MΦs plus connective tissue) and MΦ-rich area ( Supplementary Fig. 9 ). In contrast to the development of atherosclerosis in the aortic root, plaque formation in the abdominal aorta is heterogeneous and covers a length of 2 cm, which excludes histological analysis for an accurate assessment. Instead, we performed longitudinal in vivo 9.4 T MRI in a subset of mice ( N =40, 7–9 per group, Supplementary Fig. 10 ). Examples of histological sections of the abdominal aorta are displayed in Supplementary Fig. 11 . Our in vivo MRI data showed that compared with the [S]-rHDL-treated group vessel wall thickness was 16% higher in the placebo group (Mann–Whitney U -test P =0.01), 12% higher in the oral statin group (Mann–Whitney U -test P =0.004) and 16% higher in the rHDL group (Mann–Whitney U -test P =0.005, Fig. 4a,b ) at the end of the study. 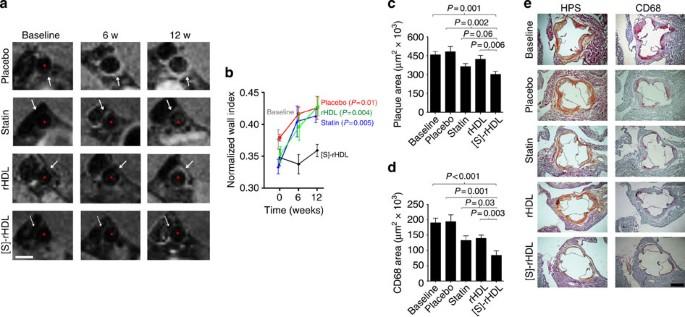Figure 4:In vivoefficacy of 12 weeks biweekly low-dose [S]-rHDL infusions. (a) Efficacy of [S]-rHDL on abdominal atherosclerosis quantified by 9.4 Tesla MRI (9.4T-MRI). Typical T1-weighted MR images of the abdominal aortas of mice in each group at all time points show the thickening of the aorta wall in all groups except in the [S]-rHDL-treated group. The analysis method of the images is shown inSupplementary Fig. 9. The scale bar represents 1 mm. (b) MRI scans of the abdominal aortas of 32 mice (N=8 per group) were performed at three time points during the study. When the apoE-KO mice were 14 weeks on high-cholesterol diet, the baseline scans were acquired and subsequent scans were performed 6 and 12 weeks after the baseline scan. From baseline onwards, the mice received placebo, oral statin therapy or injections of rHDL or [S]-rHDL. Thickness of the vessel wall is expressed as the NWI, which is defined as the ratio between the mean wall area and the outer wall area. (c) Efficacy of [S]-rHDL assessed with histology shows that the mean plaque area was lower in the [S]-rHDL-treated group (N=15) as compared with placebo (N=16) and rHDL (N=16), and there was a trend towards decreased plaque area compared with statin therapy (N=15). Kruskal–WallisP-value for plaque area is 0.0011. (d) Plaque macrophage content as measured by the CD68-positive area was decreased in the [S]-rHDL group (N=15) as compared to placebo- (N=16), statin- (N=15) and rHDL therapies (N=16), indicating decreased plaque inflammation in the [S]-rHDL group. Bars represent the s.e.m.,P-values were calculated with Mann–WhitneyU-tests. Kruskal–WallisP-value for CD68 area is 0.0001. (e) Typical histology images of the aortic sinus area of each group are shown. The HPS-stained images are shown on the left and the cross-sections stained with CD68 antibodies are shown on the right. The analysis method of the histology images is shown inSupplementary Fig. 9. The scale bar represents 400 μm. Figure 4: In vivo efficacy of 12 weeks biweekly low-dose [S]-rHDL infusions. ( a ) Efficacy of [S]-rHDL on abdominal atherosclerosis quantified by 9.4 Tesla MRI (9.4T-MRI). Typical T1-weighted MR images of the abdominal aortas of mice in each group at all time points show the thickening of the aorta wall in all groups except in the [S]-rHDL-treated group. The analysis method of the images is shown in Supplementary Fig. 9 . The scale bar represents 1 mm. ( b ) MRI scans of the abdominal aortas of 32 mice ( N =8 per group) were performed at three time points during the study. When the apoE-KO mice were 14 weeks on high-cholesterol diet, the baseline scans were acquired and subsequent scans were performed 6 and 12 weeks after the baseline scan. From baseline onwards, the mice received placebo, oral statin therapy or injections of rHDL or [S]-rHDL. Thickness of the vessel wall is expressed as the NWI, which is defined as the ratio between the mean wall area and the outer wall area. ( c ) Efficacy of [S]-rHDL assessed with histology shows that the mean plaque area was lower in the [S]-rHDL-treated group ( N =15) as compared with placebo ( N =16) and rHDL ( N =16), and there was a trend towards decreased plaque area compared with statin therapy ( N =15). Kruskal–Wallis P -value for plaque area is 0.0011. ( d ) Plaque macrophage content as measured by the CD68-positive area was decreased in the [S]-rHDL group ( N =15) as compared to placebo- ( N =16), statin- ( N =15) and rHDL therapies ( N =16), indicating decreased plaque inflammation in the [S]-rHDL group. Bars represent the s.e.m., P -values were calculated with Mann–Whitney U -tests. Kruskal–Wallis P -value for CD68 area is 0.0001. ( e ) Typical histology images of the aortic sinus area of each group are shown. The HPS-stained images are shown on the left and the cross-sections stained with CD68 antibodies are shown on the right. The analysis method of the histology images is shown in Supplementary Fig. 9 . The scale bar represents 400 μm. Full size image Subsequently, all mice ( N =74) were killed and atherosclerotic burden was quantified by means of histology of the aortic sinus. Total plaque area in the [S]-rHDL group was significantly decreased by 34% compared with the baseline group (Mann–Whitney U -test P <0.001), by 37% compared with placebo (Mann–Whitney U -test P =0.002) and by 28% compared with rHDL (Mann–Whitney U -test P =0.006, Fig. 4c ). The [S]-rHDL group showed a trend towards a decrease of 17% compared with the oral statin group (Mann–Whitney U -test P =0.06, Fig. 4c ). Plaque MΦ content was markedly decreased in the [S]-rHDL group by 56% compared with the baseline group (Mann–Whitney U -test P <0.001), by 57% compared with placebo (Mann–Whitney U -test P =0.001), by 37% compared with oral statin (Mann–Whitney U -test P =0.003) and by 40% compared with rHDL (Mann–Whitney U -test P =0.03, Fig. 4d ). In Fig. 4e , typical and representative histological sections of the different groups are shown. We also quantified the cholesterol content of the thoracic aortas of all mice ( N =74), by digesting the excised aortas followed by chemical quantification of the cholesterol content. In line with expectation, we did not observe any differences in aorta cholesterol content across all groups ( Supplementary Fig. 12 ). Serum triglyceride and total cholesterol levels did not differ significantly across all groups, although total cholesterol had the tendency to be higher in the placebo and rHDL groups ( Supplementary Fig. 13 ). Total cholesterol levels were equal in the oral statin and [S]-rHDL groups; however, fast-performance liquid chromatography showed that the oral statin group had a more favourable lipid profile than the [S]-rHDL group, with 31% lower very low-density lipoprotein, 16% lower LDL and 37% higher HDL cholesterol ( Supplementary Fig. 14 ). The decrease in plaque MΦ area by [S]-rHDL remained significant compared with placebo (multiple linear regression analysis P =0.002), oral statin (multiple linear regression analysis P =0.01) and rHDL (multiple linear regression analysis P =0.02) after statistical adjustment for serum total cholesterol levels. In vivo efficacy of high-dose [S]-rHDL infusions To assess the effect of short-term high-dose [S]-rHDL therapy on plaque inflammation, apoE-KO mice that had developed advanced atherosclerotic lesions after 27 weeks of the high-cholesterol diet were administered high-dose [S]-rHDL (60 mg kg −1 statin, 40 mg kg −1 ApoA1, N =7), placebo (saline infusion, N =15), high-dose rHDL (40 mg kg −1 ApoA1, N =8) or low-dose [S]-rHDL (15 mg kg −1 statin, 10 mg kg −1 ApoA1, N =10). All mice ( N =40) received four infusions of their assigned therapy within a single week. Histological assessment of the aortic sinus area was performed as described before ( Supplementary Fig. 9 ), and a total of 1,680 cross-sections were analysed. Histology showed a trend towards a decrease of 31% in total plaque area in the high-dose [S]-rHDL group compared with placebo (Mann–Whitney U -test P =0.053), and was decreased by 34% compared with high-dose rHDL (Mann–Whitney U- test P =0.005) and by 36% compared with the low-dose [S]-rHDL group (Mann–Whitney U- test P =0.006, Fig. 5a ). The decrease in total plaque area primarily accounted for the decreased MΦ-positive areas in the high-dose [S]-rHDL group. It was decreased by 84% when compared with placebo (Mann–Whitney U- test P <0.001), by 79% compared with high-dose rHDL (Mann–Whitney U- test P =0.001) and by 77% compared with low-dose [S]-rHDL (Mann–Whitney U- test P =0.002, Fig. 5b ). In Fig. 5c , typical and representative histological sections of the different groups are shown. Serum triglyceride and total cholesterol levels were equal across all the groups ( Supplementary Fig. 15 ). The difference in plaque MΦ content between the [S]-rHDL group and placebo (multiple linear regression analysis P <0.001), oral statin (multiple linear regression analysis P <0.001) and rHDL (multiple linear regression analysis P =0.004) remained significant after statistical adjustment for serum total cholesterol levels. 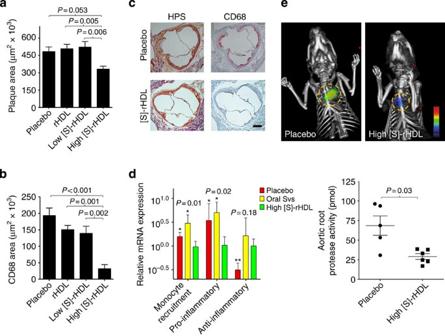Figure 5:In vivoefficacy of a single week high-dose [S]-rHDL infusions. (a) The mean plaque area was lower in the high-dose [S]-rHDL-treated group (N=10) as compared with placebo (N=15), high-dose rHDL (N=8) and low-dose [S]-rHDL (N=10). Kruskal–WallisP-value for plaque area is 0.037. (b) Plaque macrophage content as measured by the CD68-positive area was decreased in the high-dose [S]-rHDL (N=10) as compared with placebo (N=15), high-dose rHDL (N=8) and low-dose [S]-rHDL (N=10), indicative of decreased plaque inflammation in this group. Bars represent the s.e.m.,P-values were calculated with Mann–WhitneyU-tests. Kruskal–WallisP-value for CD68 area is 0.0006. (c) Typical histology images of the aortic sinus area from a mouse in the placebo group and a mouse in the high-dose [S]-rHDL group show that the mean plaque area is similar, while the plaque macrophage content is notably smaller in the [S]-rHDL group. The HPS-stained images are shown on the left and the cross-sections stained with CD68 antibodies are shown on the right. The scale bar represents 400 μm. (d) One-week high-dose [S]-rHDL treatment (N=6) significantly reduced the mRNA expression levels of monocyte recruitment genes (composite variable of MCP-1, CCL-3, ICAM-1, VCAM-1, CCL-15 and CXCL-12) and pro-inflammatory genes (composite variable of TNF-α, IL-1β, IL-1α and SPP-1) of plaque macrophages in the aortic root when compared with placebo (N=6) and oral statin (N=6). The expression of the anti-inflammatory mRNA level (MR) was increased in the high-dose [S]-rHDL group as compared with placebo but not compared with oral statin therapy.P-values are calculated with Mann–WhitneyU-tests for comparisons with [S]-rHDL, *P<0.05, **P<0.01. Kruskal–WallisP-values are shown in the plot. The error bars represent the s.d. (e) FMT-CT molecular imaging of protease activity revealed that high-dose [S]-rHDL treatment (N=6) significantly reduced the inflammation levels in the aortic roots of live apoE-KO mice with advanced atherosclerosis as compared with placebo (N=5). The yellow circles indicate the aortic root area. The error bars represent the s.e.m.P-values were calculated with the Mann–WhitneyU-test. Figure 5: In vivo efficacy of a single week high-dose [S]-rHDL infusions. ( a ) The mean plaque area was lower in the high-dose [S]-rHDL-treated group ( N =10) as compared with placebo ( N =15), high-dose rHDL ( N =8) and low-dose [S]-rHDL ( N =10). Kruskal–Wallis P -value for plaque area is 0.037. ( b ) Plaque macrophage content as measured by the CD68-positive area was decreased in the high-dose [S]-rHDL ( N =10) as compared with placebo ( N =15), high-dose rHDL ( N =8) and low-dose [S]-rHDL ( N =10), indicative of decreased plaque inflammation in this group. Bars represent the s.e.m., P -values were calculated with Mann–Whitney U -tests. Kruskal–Wallis P -value for CD68 area is 0.0006. ( c ) Typical histology images of the aortic sinus area from a mouse in the placebo group and a mouse in the high-dose [S]-rHDL group show that the mean plaque area is similar, while the plaque macrophage content is notably smaller in the [S]-rHDL group. The HPS-stained images are shown on the left and the cross-sections stained with CD68 antibodies are shown on the right. The scale bar represents 400 μm. ( d ) One-week high-dose [S]-rHDL treatment ( N =6) significantly reduced the mRNA expression levels of monocyte recruitment genes (composite variable of MCP-1, CCL-3, ICAM-1, VCAM-1, CCL-15 and CXCL-12) and pro-inflammatory genes (composite variable of TNF-α, IL-1β, IL-1α and SPP-1) of plaque macrophages in the aortic root when compared with placebo ( N =6) and oral statin ( N =6). The expression of the anti-inflammatory mRNA level (MR) was increased in the high-dose [S]-rHDL group as compared with placebo but not compared with oral statin therapy. P -values are calculated with Mann–Whitney U -tests for comparisons with [S]-rHDL, * P <0.05, ** P <0.01. Kruskal–Wallis P -values are shown in the plot. The error bars represent the s.d. ( e ) FMT-CT molecular imaging of protease activity revealed that high-dose [S]-rHDL treatment ( N =6) significantly reduced the inflammation levels in the aortic roots of live apoE-KO mice with advanced atherosclerosis as compared with placebo ( N =5). The yellow circles indicate the aortic root area. The error bars represent the s.e.m. P -values were calculated with the Mann–Whitney U -test. Full size image In a subsequent study, also in apoE-KO mice ( N =36) with advanced atherosclerosis, we determined the mRNA expression levels of genes related to inflammation in plaque MΦs by means of laser capture microdissection (LCM). We compared mice treated with high-dose [S]-rHDL with mice treated with oral statin therapy and placebo ( Fig. 5d , Supplementary Fig. 16 ). We observed that in the high-dose [S]-rHDL group, mRNA expression levels of Mo-recruitment genes ( MCP-1 , CCL-3 , ICAM-1 , VCAM-1 , CCL-15 and CXCL-12 ), as well as those of pro-inflammatory genes ( TNF-α , IL-1β , IL-1α and SPP-1 ), were markedly decreased as compared with the oral statin and placebo groups ( Fig. 5d ). The anti-inflammatory mannose receptor (MR) mRNA level was increased in the high-dose [S]-rHDL group as compared with placebo but was similar to the oral simvastatin group ( Fig. 5d ). Finally, to corroborate these findings we performed in vivo fluorescence molecular tomography with computed tomography (FMT-CT) imaging to visualize and measure the protease activity in the aortic roots of another 11 apoE-KO mice. We revealed that the inflammatory protease activity was markedly reduced in apoE-KO mice treated with [S]-rHDL as compared with placebo ( Fig. 5e ). Together, these data demonstrate the potent local anti-inflammatory effect of [S]-rHDL in atherosclerotic plaques. In the current study, we described the development of a statin-rHDL nanoparticle as a therapy for reducing atherosclerotic plaque inflammation. The key findings of our study are that this compound (1) suppresses the inflammatory response of MΦs, which is mediated through the inhibition of intracellular mevalonate pathway, (2) accumulates in atherosclerotic plaque where it is taken up by MΦs, (3) markedly reduces plaque MΦ content and inflammation following both prolonged low-dose therapy as well as short-term high-dose therapy and (4) does not exhibit myo- or hepatotoxic effects. The platform on which we based our nanoparticle is rHDL. Traditionally, HDL is considered to remove excess cholesterol from peripheral tissues and transport it to the liver for faecal excretion, a process referred to as the ‘reverse cholesterol transport’ [21] , [22] . For this reason, previous studies have investigated rHDL as a therapeutic agent. Shah et al . [23] showed that in apoE-KO mice, 18 infusions of 40 mg kg −1 ApoA1 within 5 weeks had no effect on plaque size but reduced plaque lipid content by 40% and plaque MΦ content by 46%. In another study, Shah et al . [24] showed in apoE- KO mice that a single injection of 400 mg kg −1 ApoA1 reduced plaque lipid content by 40–50% and plaque MΦ content by 29–36%. It is important to note that in the current study we did not aim at employing rHDL or ApoA1 as a therapeutic agent, apart from its ability to deliver statin to plaque tissue. Compared with the studies by Shah et al . [24] , we used lower ApoA1 doses, namely 24 infusions of 10 mg kg −1 in the 3-month low-dose study and four infusions of 40 mg kg −1 ApoA1 in the single-week high-dose study. In both our low- and high-dose studies, plaque size was unchanged in the rHDL group as compared with placebo; however, plaque MΦ content tended to be lower in the rHDL groups as compared with placebo. Despite this, we were able to show a marked reduction in plaque MΦ content by [S]-rHDL treatment compared with the rHDL group. rHDL infusion has also been investigated in large randomized controlled trials in humans [25] , [26] . Although the therapeutic efficacy was disappointing, the ApoA1 doses of 40 mg kg −1 used in these studies were well tolerated. This shows that the ApoA1 doses of 10 and 40 mg kg −1 that we used can safely be translated to future human studies. In addition to the ability of HDL to remove excess cholesterol from atherosclerotic plaques, native HDL also transports proteins involved in inflammation, coagulation, complement activation [27] and endogenous micro RNAs, and delivers them to recipient cells [28] . This indicates that native HDL is in fact a carrier vehicle involved in complex intercellular communication. In the current study, we utilize this natural property of HDL to act as a delivery vehicle of statins to target MΦs in atherosclerotic lesions. We showed that rHDL protects the statin cargo from catabolism in the serum, increases the bioavailability of statin and delivers its cargo to plaques where it is taken up by plaque MΦs. Our data on pharmacokinetics demonstrate that in the circulation [S]-rHDL is predominantly located in the plasma and a small subfraction is located in blood Mos. Blood Mos that took up [S]-rHDL in the circulation and subsequently infiltrated the plaque could potentially account for some of the accumulation of [S]-rHDL in the plaque. However, direct infiltration from the plasma into the plaque most likely accounts for the majority of [S]-rHDL accumulation in plaques. The reason why, within the vasculature, [S]-rHDL preferentially accumulates at sites of atherosclerotic lesions is likely related to local endothelial permeability, which facilitates infiltration of the nanoparticle into the vascular tissue, after which it is retained because of ingestion by MΦs. We did not investigate the mechanism by which plaque MΦs take up [S]-rHDL. Native HDL is known to interact with MΦs through scavenger receptor B1 and adenosine triphosphate-binding cassette transporters A1 and G1 (refs 21 , 22 ). Possibly our nanoparticle has a similar interaction or is simply phagocytosed by MΦs. The current study is the first to pursue local delivery of statins to plaque tissue to achieve local anti-inflammatory effects. The immunomodulating effects of statins have been established in previous studies, which showed that HMGR inhibition reduces the production of downstream isoprenoid intermediates (for example, farnesyl pyrophosphate) in the intracellular cholesterol synthesis pathway, which decreases the isoprenylation of proteins [29] , [30] . This interferes with the attachment of proteins to the cell membrane, which affects proliferation and function of inflammatory cells, such as MΦs [9] , [10] , [11] . In the current study, we confirm the anti-inflammatory effect of statins both in vitro and in vivo . In vitro , we show that the anti-inflammatory effect remains equally potent when statin is encapsulated in rHDL as compared with free statin. We also demonstrate that the anti-inflammatory effects of statins are mediated through the inhibition of the mevalonate pathway, which corroborates the results from previous studies [9] , [10] , [11] . A previous study in an atherosclerotic mouse model investigated the effects of oral statin therapy on atherogenesis. Sparrow et al . [12] treated apoE-KO mice daily with 100 mg kg −1 simvastatin for 6 weeks and showed marked reduction in aortic plaque development, despite the fact that statin therapy did not affect serum lipid levels. They also showed effects of their high-dose oral statin therapy on carrageenan-induced footpad oedema, a model of inflammation. They did not investigate the mechanism by which atherogenesis and inflammation was reduced; however, it is conceivable that higher than normal serum levels of statins were achieved since their oral statin dose was extremely high. In humans it is not possible to administer such high oral doses because of adverse effects [13] . In the current study, we used a lower oral statin dose than that used by Sparrow et al . [12] , namely 15 mg kg −1 in the 3-month low-dose study. Plaque size and MΦ content tended to be lower in the oral statin group compared with placebo. Nonetheless, we showed a marked reduction in plaque inflammation with [S]-rHDL treatment, despite 3.5 times lower weekly doses of statin in the [S]-rHDL group (15 mg kg −1 simvastatin, two times per week) than that in the oral statin group (15 mg kg −1 simvastatin per day). In addition to the decrease in plaque MΦ content following [S]-rHDL treatment, we were able to show that [S]-rHDL markedly affects plaque MΦ mRNA expression levels of genes related to inflammation. Furthermore, we observed that short-term high-dose [S]-rHDL treatment markedly decreased inflammatory protease activity in atherosclerotic plaques, which was measured in vivo with FMT-CT. Of note, in the current study we focused on the anti-inflammatory effect of our nanoparticle, since statins do not affect serum lipid levels in this mouse model. However, we showed that in mice, nanoparticles were taken up in the liver. In humans, [S]-rHDL will undoubtedly also be taken up by hepatocytes, where the delivered statin will upregulate the LDL-receptor expression. Thus, in humans, our nanoparticle may have two therapeutic effects, namely an anti-inflammatory effect on plaques and a cholesterol-lowering effect because of its affect on hepatocytes. The clinical implications of our findings pertain to the field of cardiovascular disease. With current standard of care therapy, recurrent angina before discharge occurs in up to 10% of patients following an acute coronary syndrome and recurrent acute coronary syndrome within the first year in 17.4% of patients [3] . Therefore, novel therapeutic strategies such as rHDL infusion are being developed, with the concept to initiate therapy directly after the acute event in an effort to rapidly decrease plaque vulnerability. Unfortunately, the efficacy of rHDL infusion alone so far has been disappointing [25] , [26] . Extrapolating from the evidence provided, we envision that [S]-rHDL nanotherapy can facilitate plaque retention of high quantities of statin following short-term i.v. administration in acute coronary syndrome patients, thereby modulating plaque inflammation [31] . This holds promise to suppress plaque inflammation during the vulnerable period following acute coronary syndrome, which can support the standard-of-care therapy to prevent recurrent plaque rupture and atherothrombotic events. An advantage of nanotherapy we present is that the individual components are well tolerated by humans. Statins are prescribed routinely to millions of patients worldwide, whereas rHDL in lower concentrations has proven to be safe in large phase IIB trials [13] , [25] , [26] . In our study, we did not observe myo- or hepatotoxicity of our nanoparticle. Therefore, [S]-rHDL represents a novel anti-atherosclerotic nanotherapy with a high potential for clinical translation. In conclusion, [S]-rHDL nanotherapy locally treats atherosclerotic inflammation at the level of the vessel wall. The potency of the treatment allows for the inhibition of plaque inflammation using a long-term, low-dose treatment regimen, while a short-term, high-dose treatment regimen can be applied to rapidly prevent inflammation in advanced atherosclerotic plaques. Synthesis of [S]-rHDL The synthesis of [S]-rHDL was modified from a published method [32] . Briefly, simvastatin (AKscentific), 1-myristoyl-2-hydroxy-sn-glycero-phosphocholine and 1, 2-dimyristoyl-sn-glycero-3-phosphatidylcholine (both purchased from Avanti Polar Lipids) were dissolved in chloroform/methanol (4:1 by volume) solvent and dried to form a thin film. Human ApoA1 (CSL, Parkville, Victoria, Australia) dissolved in phosphate-buffered saline (PBS) were added to the film and the solution was incubated in 37 °C until the film was hydrated and a homogenous solution was formed. The solution was sonicated to form small [S]-rHDL nanoparticles. Aggregates were removed using centrifugation and filtration. Gadolinium–DTPA–DMPE (Avanti Polar Lipids), Cy5.5-DMPE (DMPE was conjugated with Cy5.5 NHS–ester purchased from GE Healthcare), DiR or DiO (Invitrogen) were added when the nanoparticles were subsequently used for imaging purposes. Control rHDL nanoparticles without simvastatin were synthesized with the same procedures. Characterization of [S]-rHDL Nanoparticles were negatively stained with a method previously reported [33] . Briefly, samples were suspended in an ammonium acetate buffer using a 2% sodium phosphotungstate (pH=7.4) negative stain. The mixed solution were subsequently added to TEM grids, dried, and finally subjected to TEM imaging. Images were acquired using a Hitachi H7650 system linked to a Scientific Instruments and Applications digital camera controlled by the Maxim CCD software. The mean size of the different formulations of nanoparticles was determined by dynamic light-scattering (Brookhaven Instruments Corporation, Holtsville, NY, USA) and by measuring the nanoparticles in TEM images. The percentage of phospholipids in the nanoparticles was determined by Rouser’s method; the percentage of simvastatin by HPLC (Shimadzu HPLC instrument); the percentage of protein by a BCA protein concentration assay (Bio-Rad); the longitudinal relaxivity (r1) of gadolinium-loaded [S]-rHDL was measured on a 60-MHz Bruker Minispec (Bruker Medical BmbH, Ettingen) operating at 40 °C. To determine the half-life of encapsulated simvastatin in [S]-rHDL, a concentration of 1,000 μg ml −1 of simvastatin from [S]-rHDL or free simvastatin was achieved in mouse serum and the solution was kept at 37 °C. The concentration of intact simvastatin in the serum at different time points was measured with HPLC (Shimadzu HPLC equipped with a column (Ascentis C18, 10 cm × 4.6 mm I.D., 3 μm particles (581321-U) reversed phase)) using a protocol adapted from the published one [34] . The mobile phase was 80% Acetonitrile and 20% H 2 O and the flow rate was 0.5 ml min −1 . The half-life of simvastatin in [S]-rHDL and free simvastatin was defined as the length of incubation time when the serum simvastatin concentration was 500 μg ml −1 . In vitro cell assays J774A.1 (murine MΦs), MS1 (murine endothelial cells), MOVAS (murine aortic smooth muscle cells) and Hepa-1c1c7 (murine liver cells) were cultured under American Type Culture Collection-recommended conditions. [S]-rHDL nanoparticles were added to the cells to reach different concentrations of simvastatin in cell culture, whereas rHDL nanoparticles were added to reach the same ApoA1 concentrations as [S]-rHDL under each condition, and mevalonate was added to reach 100 μM when needed. The cell viability was determined by measuring intracellular ATP concentration by following the manufacturer’s instructions (Promega, CellTiter Glo). To measure MCP-1 and TNF-α production by J774A.1 cells, the cells were first challenged with lipopolysaccharide and interferon-γ for 16 h, and subsequently switched to serum-free culture condition and treated with [S]-rHDL, free simvastatin, rHDL or nothing for another 24 h at the concentration of 10 μM simvastatin or equal concentration of ApoA1 from rHDL, in the presence or absence of 100 μM mevalonate. TNF-α and MCP-1 concentrations in the supernatants were measured with enzyme-linked immunosorbent assay by following the manufacturer’s instructions (Biolegend). For apoptosis/necrosis assay, murine cells (J774A.1) were treated with 10 μM simvastatin equivalent [S]-rHDL for 24 h, and then stained with either apoptosis-specific dye (YO-PRO-1) or necrosis-specific dye (Propidium iodide). Measurement was used following the manufacturer’s instruction (Life Technologies, Cat no. V13243). In brief, apoptotic cells are defined as YO-PRO-1-positive, Propidium iodide-positive cells on flow cytometry graph, while necrosis cells are YO-PRO-1-negative Propidium iodide-positive. For cell proliferation, an assay was performed following the manufacturer’s instruction (Life Technologies, Cat no. C34554). In brief, MΦs were incubated with 5 μM carboxyfluorescein succinimidyl ester (CFSE) for 10 min and the rest of the CFSEs were extensively removed. Subsequently, the cells were treated with 10 μM simvastatin equivalent [S]-rHDL or nothing for 24 h. The percentage of proliferating cells of the total treated cells was determined using flow cytometry following a standard protocol. Animals and diet All animals were used based on an approved institutional protocol from the Icahn School of Medicine at Mount Sinai. Five-week-old male apoE-KO mice (B6.129P2-Apoe tm1Unc ) were purchased from Jackson laboratory. All mice were fed with a high-cholesterol diet, containing 20.3% fat, 22.9% protein, 45.7% carbohydrate and 0.2% cholesterol (Research Diets Inc., USA). In vivo 9.4 Tesla MRI To image the abdominal aortas, the mice were anaesthetized and maintained by isoflurane-containing air and were subsequently scanned with a 9.4 Tesla MRI system (Bruker Instruments, Germany). T1-weighted MRI was performed using a black blood sequence. Twenty-two consecutive 500-μm-thick slices with 500 μm inter-slice distance were acquired using a spin echo sequence with a 256 × 256 matrix size. A microscale in-plane resolution of 101 μm was achieved. The repetition time and echo time for the T1-weighted scanning were 800 and 8.6 ms, respectively. An inflow saturation band of 3 mm was used with a slice gap of 3 mm for additional luminal flow suppression. Sixteen signal averages were used for a total imaging time of 55 min per scan. A saturation pulse was used to eliminate signal from fat tissue and to delineate boundary of the aortic wall and minimize chemical shift artifacts. To investigate the plaque targeting of [S]-rHDL, the mice were first subjected to baseline MRI scan, and subsequently injected with a 50-μmol Gadolinium kg −1 dose of the [Gd-S]-rHDL through their tail veins. The mice were scanned again at 24 h post injection ( N =3). Image analysis was performed with a semiautomatic software (VesselMass, Leiden) to delineate the aortic lumen area and outer wall area (OWA). The mean wall area (MWA) was defined as the difference between lumen area and OWA. The primary outcome parameter was the normalized wall index (NWI), which was calculated as: NWI=MWA/OWA. To evaluate the therapeutic effects of 12-week treatments, mice were scanned with the same protocol but without the injection of contrast agents. Ex vivo NIRF The mice were injected with Cy5.5-DMPE- and DiR-labelled [S]-rHDL ( N =3) or saline ( N =3) through their tail veins. At 24 h post injection, mice were killed and perfused with PBS. To acquire Cy5.5 signal from [S]-rHDL in tissues, aortas, hearts, livers, spleens and kidneys were collected and imaged with IVIS 200 system (Xenogen) using 675(30) nm excitation and 720 (20) nm emission filters. Photon counts were used to quantify the fluorescence intensity from each tissue and it was reflected by colour-coded scale bar. Images were processed with the integrated software from IVIS 200 (Living Imaging Software 4.0). DiR signal was acquired with the same procedure but imaged with 745(30) nm excitation and 820 (20) nm emission filters. Flow cytometry To investigate the targeting mechanism of [S]-rHDL, apoE-KO mice were injected with Cy5.5 and DiO dual-labelled [S]-rHDL at doses of 15 mg kg −1 simvastatin and 10 mg kg −1 ApoA1, the same as the low-dose 12-week [S]-rHDL treatment. The mice were killed at individual time points post injection (1, 2, 4, 6, 12 and 24 h; N =3 per time point). Blood was collected and RBCs were lysed and removed using RBC lysis buffer (BD Biosciences). The mice were perfused with PBS and cells from aortas were collected using the same method as described above. After perfusion with 30 ml of PBS, aortas were collected and the surrounding adipose tissue was removed carefully without damaging the adventitia. Aortas were digested with 4 U ml −1 liberase LH (Roche), 0.1 mg ml −1 DNase I (Sigma-Aldrich) and 60 U ml −1 hyaluronidase (Sigma-Aldrich) in hank's balanced salt solution (HBSS) at 37 °C for 90 min. The suspension was incubated with a mixture of monoclonal antibodies for 30 min at 4 °C. Fluorescence was detected using a flow cytometer (BD Biosciences LSR II), and the data were analysed using the FlowJO software (Tree Star). MΦs from aortas were identified as CD45+, CD11b+ and F4/80+, and Mos were identified as CD45+, CD11b+ and SSC-A low cells. Based on the Gr-1 expression, Mos in the blood were further identified as Gr-1 hi and Gr-1 lo Mos. To quantify the delivery efficiency to Mos, MΦs and neutrophils in the spleen, a recently reported protocol was used [4] . Briefly, splenocytes were released by homogenizing the spleen, and the tissue was digested with collagenase (Sigma-Aldrich) for 30 min at 37 °C. A cocktail of antibodies include a Pacific blue-conjugated lineage (CD90 (clone 53-2.1), B220 (clone RA3-6B2), CD49b (clone DX5), NK1.1 (clone PK136), Ly-6G (clone 1A8) and Ter-119 (clone TER-119)), Alexa700-conjugated CD11b (clone M1/70), antigen-presenting cell-conjugated CD11c (clone HL3), phycoerythrin-Cy7-conjugated F4/80 (clone BM8) and PE-conjugated Ly6C (clone AL-21). Neutrophils were identified as Lineage high, CD11b high, ly-6c intermediate and SSC-A high. MΦs were identified as lineage−, CD11b high, and F4/80+. Mos were identified as Lineage−, CD11b high, CD11c−, F4/80− and Ly-6C+. Based on Ly-6c expression levels, Mos were further identified as Ly-6c high and Ly-6c low Mos. All antibodies were purchased from eBioscience, BD Biosciences and Biolegend, and a 1:200 dilution was used. Fluorescence quantification of blood components ApoE-KO mice received dual-labelled [S]-rHDL (Cy5.5 and DiO) through tail vein injection. At each individual time point (1, 2, 4, 6, 12 and 24 h; N =3 per time point), mouse blood was drawn with cardiac puncture and stored in EDTA-containing tubes. Blood (500 μl) was used for separating different compartments with Histopaque (Sigma-Aldrich, Histopaque 1077) by following the instructions from the manufacturer. Briefly, the blood and Histopaque solution were centrifuged at room temperature for 30 min, and three compartments from the blood (serum; MNCs; RBCs and granulocytes) were visible and collected. Fifty microlitre solution from each compartment was added to a 96-well plate (three repeats for each condition). The plate was imaged with IVIS 200 system (Xenogen). To image DiO, excitation filter of 465 (30) nm and emission filter of 520 (20) nm were used. To image Cy5.5, excitation filter of 675 (30) nm and emission filter of 720 (20) nm were used. Signal intensity was analysed and quantified using the integrated software from the system (Living Imaging Software 4.0). Immunohistochemistry and image quantification Serial 6 μm thick cross-sections were made of the aortic sinus area on a cryotome (Reichert HistoStat, Cryostat Microtome). From the first cross-section in which the leaflets of the aortic valves appeared upward, 63 serial cross-sections were obtained, covering the entire aortic sinus area. Every three consecutive cross-sections were subjected to anti-CD68 immunohistochemical staining, HPS staining, and Oil Red O staining. HPS (HPS, polyscientific) and Oil Red O staining (Fisher Scientific) were performed with the standard methods. For anti-CD68 staining, the sections were blocked with rabbit serum (Vectorlabs), incubated for 1 h with rat anti-mouse CD68 primary antibody (Abdserotec, 1:250 dilution), for 10 min with biotinylated rabbit anti-rat antibody (Vectorlabs, 1:200 dilution), for 5 min with VECTASTAIN ABC-alkaline phosphatase solution (Vectorlabs) and finally for 17 min with Vector Red solution (Vectorlabs). All the cross-sections were digitally imaged with a Nikon eclipse E400 microscope, with a × 10 eyepiece and × 10 lenses, a Nikon DS-U1 camera box and Nikon DS-5M camera. We used the NIS-Elements F3.0 software and imaged the cross-sections at a 1/350-s exposure time, 2,560 × 1,920 pixels and pixel size of 1.46 μm 2 per pix. Software written in Matlab was developed to facilitate automated image analysis. Treatment protocol For the 12 weeks of treatment study, 6-week-old male apoE-KO mice were fed a high-cholesterol diet (ResearchDiets, NJ) for 14 weeks and subsequently received 12 weeks of i.v. injection of [S]-rHDL (15 mg kg −1 simvastatin, 10 mg kg −1 ApoA1, 2 injections per week, N =16) and rHDL (10 mg kg −1 ApoA1, 2 injections per week, N =16), and oral administration of simvastatin (15 mg kg −1 per day, two saline i.v. injections per week, N =15) and placebo (two saline injections per week, N =15). Mice were maintained on a high-fat diet during the 12-week treatment. Another group of mice ( N =12) was killed when the other groups started their 12-week treatment to establish a baseline. Eight mice per group were imaged with MRI over abdominal aortas before, in the middle and by the end of the 12-week treatments. For the 1-week short-term treatment study, 6-week-old male apoE-KO mice were fed a high-cholesterol diet for 27 weeks. After the diet, mice were injected intravenously with high-dose [S]-rHDL (60 mg kg −1 simvastatin, 40 mg kg −1 ApoA1 and four injections per week), high-dose rHDL (40 mg kg −1 ApoA1, four injections per week), low-dose [S]-rHDL (15 mg kg −1 simvastatin, 10 mg kg −1 ApoA1 and four injections per week) or placebo (four saline injections per week). Laser capture microdissection and qRT–PCR Thirty-six 6-week-old male apoE-KO mice were fed a high-fat diet for 26 weeks to develop advanced atherosclerosis. The animals received 1-week treatment of high-dose [S]-rHDL (four i.v. infusions of 60 mg kg −1 statin, 40 mg kg −1 ApoA1, denoted as ‘high [S]-rHDL), rHDL (two i.v. infusions of 10 mg kg −1 ApoA1, denoted as ‘rHDL’), oral statin treatment (15 mg kg −1 per day oral simvastatin, denoted as ‘Oral SVS’), rHDL plus oral statin (15 mg kg −1 per day oral simvastatin and two i.v. infusions of 10 mg kg −1 ApoA1, denoted as ‘rHDL+Oral SVS’) or placebo (four i.v. injections of PBS). Sections from aortic roots were prepared as described above, and a total of 24 sections were made per animal. For every eight consecutive sections, the first one was stained with CD68 with the same method described above and was used as the guiding section. The other seven sections were used for isolating MΦs using LCM as previously described [35] . Briefly, the sections were fixed in 70% ethanol for 1 min, washed in H 2 O, stained with Mayer’s haematoxylin (VWR Scientific) for 1 min, washed in H 2 O, incubated in PBS (to develop blue colour) for 15 s, washed in H 2 O, partially dehydrated in 70% followed by 95% ethanol, stained in eosin Y (VWR Scientific) for 5 s, washed in 95% ethanol and completely dehydrated in 100% ethanol (30 s), xylene (30 s) and xylene (5 min). After air-drying for 10 min, MΦs were identified under a microscope and were verified by the CD68 staining on the guiding slides. Several hundred MΦs per mouse were collected, and these MΦs from each animal were used to extract and amplify RNA with WT-Ovation Pico RNA amplification system (NuGen). The quality of extracted RNA was measured using Agilent 2100 Bioanalyzer. Quantitative reverse transcriptase PCR (qRT–PCR) was performed on samples using the iScript cDNA Synthesis kit (Bio-Rad) according to the manufacturer’s protocol. The mRNA expression levels of investigated genes were normalized to the housekeeping gene hprt1 (UniGene ID: Mm.1037830, Assay ID: Mm01545399). The following genes were investigated: MCP-1 (Mm.290320, Mm00441242_m1), CCL-3 (Mm.1283), ICAM-1 (Mm.435508, Mm00516023_m1), VACM-1 (Mm.440909, Mm01320970_m1), CXCL-12 (Mm.303231, Mm00445553_m1), CCL-15 (Mm.284248, mm01302427_m1), TNF-α (Mm.1293, mm00443260_g1), IL-1β (Mm.222830, mm00434228_m1), IL-1α (Mm.15534, Mm00439620_m1), Spp-1 (Mm.288474, Mm00436767_m1) and MR (Mannose Receptor, Mm2019, Mm00485148_m1). TaqMan Gene Expression assay (Life Technologies, Cat no. 4331182, applied to all aforementioned genes) was used to measure the gene expression on sequence detection device (ABI PRISM 7900HT). Fluorescence molecular tomography with CT Eleven 6-week-old apoE-KO mice were fed a high-fat diet for 20 weeks before receiving four high-dose [S]-rHDL or placebo (PBS) injections in a week. Five nanomoles of pan-cathepsin protease sensor (ProSense 680, PerkinElmer, Cat no. NEV10003) was intravenously administered along with the last i.v. injection of [S]-rHDL or PBS. Twenty-four hours later, the animals were placed in a custom-built imaging cartridge, which was equipped for isoflurane administration during imaging. Animals were first scanned with high-resolution computated tomography (CT; Inveon PET-CT, Siemens), with a continuous infusion of CT-contrast agent (isovue-370, Bracco Diagnostics) at a rate of 55 μl min −1 through a tail vein catheter. Animals were subsequently scanned with an FMT scanner (PerkinElmer) in the same cartridge. The CT X-ray source with an exposure time of 370–400 ms was operated at 80 kVp and 500 μA. Contrast-enhanced high-resolution CT images were used to localize the aortic root, which was used to guide the placement of the volume of interest for the quantitative FMT protease activity map. The CT reconstruction protocol involved bilinear interpolation, used a Shepp-Logan filter and scaled pixels to Hounsfiled units. Image fusion relied on fiducial markers and used the Osirix software (The Osirix Foundation, Geneva). Blood tests and lipoprotein analysis After 4 h of fasting, whole blood was collected in an EDTA-containing tube. Some serum was subjected to a biochemistry panel (ALX laboratories, NY) analysis to determine the blood concentrations of alanine transaminase, aspartate transaminase, creatinine, creatine kinase, cholesterol and triglyceride. The rest serum was pooled per group for lipoprotein analysis via fast-performance liquid chromatography (FPLC) (Pharmacia). For each sample, 250 μl of the plasma was applied to 2 Superose 6 columns (GE Healthcare) equilibrated and run in a buffer containing 150 mM NaCl and 15 mM EDTA in deionized water. The column flow rate was 0.7 ml min −1 . Eighty fractions were collected, and the total cholesterol concentration of each fraction was assessed using an enzymatic colorimetric assay (Wako) according to the manufacturer’s instructions. Cholesterol measurement in thoracic aorta The thoracic aortas were blotted dry and weighed. Later, they were minced and extracted with chloroform/methanol (2:1) according to the method of Folch et al . [36] The cholesterol-containing supernatant was measured (WACO diagnostics) and the total cholesterol from the aortas was calculated accordingly. Finally, the ratio of cholesterol to tissue was calculated by dividing the total cholesterol content per aorta by the weight of the aorta. Statistics Continuous variables are expressed as means±s.d., unless otherwise stated. Significance of differences was calculated by use of the nonparametric Mann–Whitney U- tests and Kruskal–Wallis tests. Multiple linear regression analysis was used to assess the association between CD68 area and the various treatment groups, with CD68 area as the response variable and treatment group as the explanatory variable, adjusting for the potential confounder serum total cholesterol. Composite variables were calculated for Mo recruitment and pro-inflammatory mRNA expression in the LCM experiment. Probability values of P <0.05 were considered significant. Statistical analyses were performed using SPSS (Statistical Package for the Social Sciences) version 17.0 and SAS package (SAS Institute Inc.). How to cite this article : Duivenvoorden, R. et al . A statin-loaded reconstituted high-density lipoprotein nanoparticle inhibits atherosclerotic plaque inflammation. Nat. Commun. 5:3065 doi: 10.1038/ncomms4065 (2014).